Directional emission from a single plasmonic scatterer Directing light emission is key for many applications in photonics and biology. Optical antennas made from nanostructured plasmonic metals are suitable candidates for this purpose but designing antennas with good directional characteristics can be challenging, especially when they consist of multiple elements. Here we show that strongly directional emission can also be obtained from a simple individual gold nanodisk, utilizing the far-field interference of resonant electric and magnetic modes. Using angle-resolved cathodoluminescence spectroscopy, we find that the spectral and angular response strongly depends on excitation position. For excitation at the nanodisk edge, interference between in-plane and out-of-plane dipole components leads to strong beaming of light. For large nanodisks, higher-order multipole components contribute significantly to the scattered field, leading to enhanced directionality. Using a combination of full-wave simulations and analytical point scattering theory we are able to decompose the calculated and measured scattered fields into dipolar and quadrupolar contributions. Optical nanoantennas have the ability to control the emission and absorption of light at the nanoscale [1] . Nanoantennas composed of metallic nanoparticles that support localized surface plasmon resonances (LSPRs) in the ultraviolet-visible-infrared part of the electromagnetic spectrum have been used to control spontaneous emission [2] , [3] , [4] , [5] , [6] and surface enhanced Raman scattering [7] , [8] , and find applications in targeted medicine [9] , [10] , solar steam generation [11] , [12] or photovoltaics [13] . In many of these applications the directionality of the plasmon scattering plays a pivotal role. The angular scattering profiles of single nanoparticle antennas are usually isotropic around the symmetry axis. To obtain strong directionality in plasmonic nanoantennas multi-element array antennas such as the Yagi–Uda geometry are used. These are composed of a locally driven feed element that is coupled to several parasitic director elements that collectively interfere in the far field [14] , giving rise to directional emission [5] , [15] , [16] , [17] , [18] , [19] , [20] . However, these array antennas are complex to design and fabricate, and have a relatively large spatial footprint. Strong directionality can also be achieved using just a single element antenna if the interference between electric dipole and higher-order multipole components can be controlled [21] , [22] , [23] , [24] , [25] , [26] , [27] , [28] . However, efficient excitation of higher-order magnetic and electric multipoles requires strong field gradients on the scale of the nanoparticle, which is difficult to obtain using plane wave excitation. Since each multipole component has its own complex vectorial near-field distribution, local excitation of the nanoantenna can enable excitation of the right combination of modes that interfere in such a way as to give strongly directional emission. Here we use a tightly focused 30 keV electron beam as local excitation source to drive the resonant electric and magnetic modes in cylindrical Au nanoantennas. The evanescent electromagnetic field about the electron trajectory provides a stable and highly localized (~10 nm) broadband source of surface plasmons that does not perturb the dielectric environment enabling spatially resolved studies of plasmonic modes over a broad spectral range in a single experiment [17] , [29] , [30] , [31] , [32] , [33] , [34] , [35] , [36] , [37] . Using angle-resolved cathodoluminescence (CL) imaging spectroscopy (ARCIS) [17] , [38] , we show that the interference between locally excited multipole components in the Au particles can give rise to strongly directional emission in a single element nanoantenna. We demonstrate that the beaming direction is directly controlled by the precise electron beam position on the nanoparticle. From the spectrally filtered angular emission distributions we detect features in the locally excited plasmon radiation fields that provide key information on the modal composition of the plasmon excitation. By combining full-wave simulations and analytical point scattering theory we are able to decompose the measured far-field radiation patterns into electric dipole, magnetic dipole and electric quadrupole contributions and show that these all contribute to the antenna’s scattering profile. CL spectra We fabricated cylindrical gold nanoparticles with diameters ranging from 50–180 nm in 5 nm steps and a height of 80 nm on a crystalline silicon substrate using a combination of electron beam lithography, thermal evaporation and lift-off. For the hyperspectral imaging measurements we raster-scan the e-beam in small steps over the disk (5 nm steps for D ≤100 nm and 7.5 nm steps for D >100 nm). Light is collected by a half-parabolic mirror placed between sample and the electron microscope pole piece and directed to a grating spectrometer equipped with a liquid nitrogen cooled CCD camera. At each excitation position we collect a spectrum in the visible/near-infrared spectral region. The integration time was 500 ms per pixel at a beam current of 0.8 nA. By integrating over all scanning pixels we also obtain the average CL spectrum for each nanodisk. The spectra are normalized to the peak intensity and corrected for background radiation from the Si substrate. 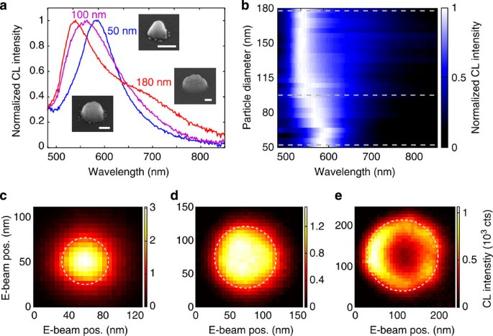Figure 1: CL spectra. (a) Spatially integrated normalized CL spectra for Au nanodisks withD=50, 100 and 180 nm. Scanning electron micrographs of the corresponding particles are shown as insets in which the scale bars represent 50 nm. (b) Integrated peak-normalized CL spectra for a range of different nanodisk diameters in 5 nm steps. The grey dashed lines indicate diameters for which spectra are shown in (a). CL intensity as function of excitation position for (c)D=50 nm atλ0=580 nm, (d)D=100 nm atλ0=560 nm and (e)D=180 nm atλ0=550 nm, integrated over a 20 nm bandwidth. Figure 1a shows spatially-averaged spectra for Au nanodisks with D =50, 100, and 180 nm, respectively. The corresponding scanning electron micrographs of the disks are shown as insets. For the D =50 nm particle we observe a LSPR peak at λ 0 =580 nm. The peak broadens and blueshifts when the diameter is increased to 100 nm. For the largest particle ( D =180 nm) the spectrum is broadened further and shows a clear shoulder at λ 0 =700 nm suggesting a second LSPR resonance. The gradual blueshift of the main peak and the emergence of a shoulder at longer wavelengths can be seen in more detail in Fig. 1b where the spatially averaged CL spectrum is shown for all measured nanodisks with diameters in the range D =50–180 nm. Figure 1: CL spectra. ( a ) Spatially integrated normalized CL spectra for Au nanodisks with D =50, 100 and 180 nm. Scanning electron micrographs of the corresponding particles are shown as insets in which the scale bars represent 50 nm. ( b ) Integrated peak-normalized CL spectra for a range of different nanodisk diameters in 5 nm steps. The grey dashed lines indicate diameters for which spectra are shown in ( a ). CL intensity as function of excitation position for ( c ) D =50 nm at λ 0 =580 nm, ( d ) D =100 nm at λ 0 =560 nm and ( e ) D =180 nm at λ 0 =550 nm, integrated over a 20 nm bandwidth. Full size image To gain further insight into the nature of the resonant modes we plot the two-dimensional (2D) spatial maps at the peak-wavelengths for the three diameters in Fig. 1a integrated over a 20 nm spectral bandwidth ( Fig. 1c–e ). As can be seen for these wavelengths, the 50 and 100 nm disks radiate most efficiently when excited in the centre, whereas the 180 nm particle radiates most strongly when excited at the edge. From our previous work, it is known that modes that are efficiently driven by the electron beam in the particle centre usually have m =0 (azimuthal) symmetry [17] , [39] , [40] and an out-of-plane oriented electric dipole moment, whereas efficient edge excitation indicates the presence of strong in-plane dipole components ( m =1), where m is the azimuthal quantum number. In the first case the vertical component of the electric field is strong in the centre while in the second case it is strong at the edge allowing strong coupling to the electron beam at those specific positions. Considering that the nanodisk diameter/height aspect ratio changes from 0.625 (50 nm diameter) to 2.25 (180 nm diameter) respectively, it is to be expected that the in-plane components become more dominant as their scattering efficiency increases for the larger nanodisks. The evolution of the CL spectrum as function of disk diameter is governed by three effects. First, for the smaller diameters the out-of-plane dipole resonance is dominant and it is known that an increase in particle size transverse to the electric dipole resonance axis leads to a stronger restoring force and thus a blue-shifted resonance. Second, following the same reasoning the in-plane electric dipole resonance redshifts because the increase in size is now along the dipole axis. Third, higher-order resonant modes become more dominant for larger particles, having an effect on the CL spectrum. Directional scattering To gain more insight into the nature of the particle resonances, we measured the far-field angular emission patterns by projecting the beam emanating from the parabolic mirror onto a 2D CCD array. The CCD data are subsequently converted to angular emission distributions [38] . We collect the angular patterns for free-space wavelenghts ( λ 0 ) from 400 to 750 nm using 40-nm band pass filters for D =50, 100, 140 and 180 nm disks. To optimize the signal-to-noise ratio, we have used 120 s integration time for λ 0 =400, 450, 700 and 750 nm and 60 s for λ 0 =500–650 nm. 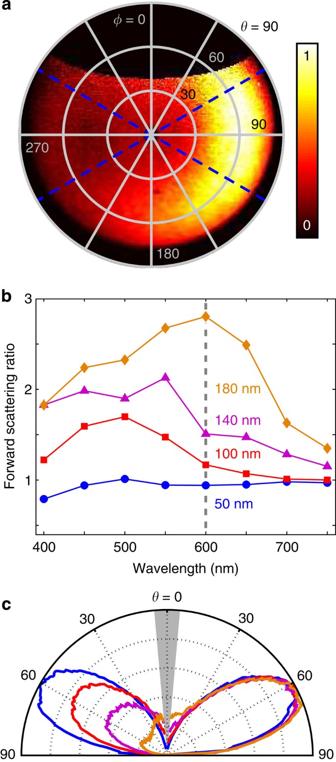Figure 2: Directional scattering. (a) Measured angular pattern for ad=180 nm nanodisk atλ0=600 nm for excitation on the left edge of the nanodisk (b) Forward scattering ratio as function of wavelength for different disk diameters. (c) Crosscuts through radiation patterns for different-diameter disks atλ0=600 nm (corresponding to the grey dashed line in (b)), plotted with the same colour code as in (b). The crosscuts have been integrated over a range ofϕ(ϕ=60–120° andϕ=270–330° as indicated by the blue dashed lines in (a)). For visibility all patterns in (c) have been normalized to 1. The grey region is not collected due to the hole in the parabolic mirror. Figure 2a shows the angular pattern for a D =180 nm particle at λ 0 =600 nm for excitation on the ‘left’ edge of the nanodisk. The pattern clearly shows a strong angular asymmetry. When excited at the edge, the particle preferentially radiates away from the excitation point. Angular patterns for four orthogonal edge positions are shown in Fig. 3 , demonstrating that the beaming is always directed away from the excitation point. If the nanodisk is excited in the centre the emission intensity is lower (also see Fig. 1e ) and an azimuthally symmetric toroidal emission pattern is observed consistent with the radiation pattern of a vertically oriented electric dipole on top of a high-index substrate. A similar beaming effect also occurs for D =100 nm disks, which is shown in Fig. 4a–c ) for λ 0 =600 nm. In contrast, for D =50 nm disks the pattern remains almost toroidal for all excitation positions and very closely matches the angular pattern of a vertical electric dipole (see Fig. 4d–f ). Figure 2: Directional scattering. ( a ) Measured angular pattern for a d =180 nm nanodisk at λ 0 =600 nm for excitation on the left edge of the nanodisk ( b ) Forward scattering ratio as function of wavelength for different disk diameters. ( c ) Crosscuts through radiation patterns for different-diameter disks at λ 0 =600 nm (corresponding to the grey dashed line in ( b )), plotted with the same colour code as in ( b ). The crosscuts have been integrated over a range of ϕ ( ϕ =60–120° and ϕ =270–330° as indicated by the blue dashed lines in ( a )). For visibility all patterns in ( c ) have been normalized to 1. The grey region is not collected due to the hole in the parabolic mirror. 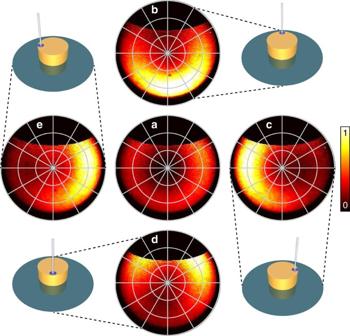Figure 3: Spatial control of angular pattern. Experimental normalized angular CL emission patterns collected from a 180 nm diameter nanodisk atλ0=600 nm for excitation at the centre (a) and near the edge for four orthogonal azimuthal angles: 0° (b), 90° (c), 180° (d) and 270° (e). The edge excitation positions are also indicated by the schematics in the corners. The patterns have been normalized to the maximum intensity value for all five patterns to show the relative brightness for different excitation positions. Full size image Figure 3: Spatial control of angular pattern. Experimental normalized angular CL emission patterns collected from a 180 nm diameter nanodisk at λ 0 =600 nm for excitation at the centre ( a ) and near the edge for four orthogonal azimuthal angles: 0° ( b ), 90° ( c ), 180° ( d ) and 270° ( e ). The edge excitation positions are also indicated by the schematics in the corners. The patterns have been normalized to the maximum intensity value for all five patterns to show the relative brightness for different excitation positions. 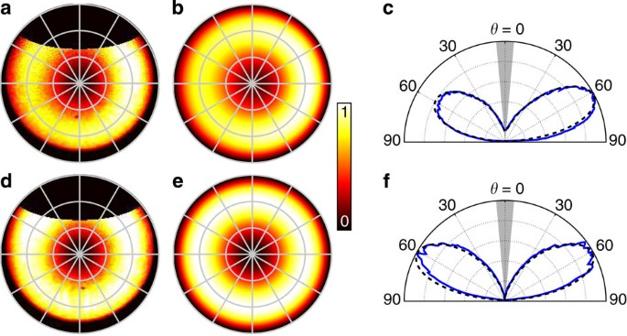Figure 4: Radiation patterns forD=100 nm andD=50 nm. (a) Measured angular emission pattern of aD=100 nm disk for left-edge excitation, measured atλ0=600 nm. Again the nanodisk beams light away from the excitation point. (b) Calculated angular pattern obtained by numerically fitting complexpzandpxdipole components (40 nm above the silicon substrate) to the data. (c) Emission intensity as function of zenithal angleθfor the experimental data from (a) (blue curve) and the theoretical pattern in (b) (black dashed curve), integrated fromϕ=60–120° andϕ=270–330° as indicated by the blue dashed lines inFig. 2a). (d) Measured angular emission pattern of aD=50 nm disk for central excitation, measured atλ0=600 nm. (e) Calculated angular pattern for a vertically oriented electric point dipole source. (f) Zenithal emission profiles for (d) and (e). Full size image Figure 4: Radiation patterns for D =100 nm and D =50 nm. ( a ) Measured angular emission pattern of a D =100 nm disk for left-edge excitation, measured at λ 0 =600 nm. Again the nanodisk beams light away from the excitation point. ( b ) Calculated angular pattern obtained by numerically fitting complex p z and p x dipole components (40 nm above the silicon substrate) to the data. ( c ) Emission intensity as function of zenithal angle θ for the experimental data from ( a ) (blue curve) and the theoretical pattern in ( b ) (black dashed curve), integrated from ϕ =60–120° and ϕ =270–330° as indicated by the blue dashed lines in Fig. 2a ). ( d ) Measured angular emission pattern of a D =50 nm disk for central excitation, measured at λ 0 =600 nm. ( e ) Calculated angular pattern for a vertically oriented electric point dipole source. ( f ) Zenithal emission profiles for ( d ) and ( e ). Full size image Figure 2b shows the magnitude of the angular asymmetry as function of wavelength, calculated from the integrated ‘forward’ and ‘backward’ half of the angular hemisphere. Data are shown for four different disk diameters. For the D =50 nm disks the measured ratio is close to 1 (except for λ 0 =400 nm), indicating that there is no asymmetry in the emission pattern. As the diameter increases, stronger angular beaming is observed and the maximum beaming condition shifts to longer wavelengths. The strongest directionality (forward-to-backward intensity ratio of 2.8) is obtained for the D =180 nm disks at λ 0 =600 nm. The increase in directionality for increasing diameter is clearly visible in Fig. 2c , which shows crosscuts through the angular data at λ 0 =600 nm for the same disk diameters as in Fig. 2b . The data in Figs 2 and 3 show that directional angular emission can be achieved from a single nanodisk by precisely positioning the local electron beam source. Note that the directionality is reversed with respect to what was shown in ref. 41 . This is due to the fact that we collect the angular patterns for the upper hemisphere, whereas in that case the patterns were measured on the substrate side where the dipole radiation ‘doughnut’ points towards the excitation point. To study the nature of the different resonant modes that contribute to the radiation patterns we study the angular emission distribution for different wavelengths. 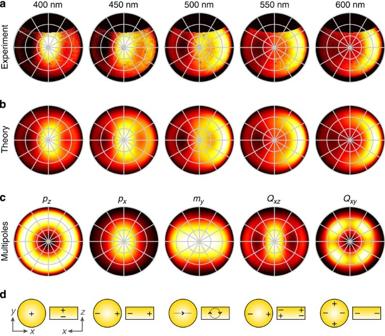Figure 5: Multipolar decomposition. Normalized experimental CL radiation patterns (row (a)) and numerically fitted theoretical patterns (row (b)) for aD=180 nm Au disk excited on the ‘left’ side forλ0=400–600 nm. The patterns are a result of the coherent interference of five multipole components. The theoretical radiation patterns for the individual components are plotted in row (c) forλ0=500 nm for a source placed 40 nm above a silicon substrate. Below each pattern the corresponding charge distribution is shown from two perspectives (row (d)): on the left, a top view of the disk and on the right, a cross section of the disk in thexzplane. Figure 5 shows normalized angular patterns for λ 0 =400–600 nm for the D =180 nm particle disk for edge excitation on the ‘left’ side. The pattern for λ 0 =400 nm shows a strong radiation lobe normal to the substrate. The relative contribution of this lobe becomes increasingly weaker for longer wavelength while the sideward lobe gradually becomes more pronounced. At λ 0 =600 nm the forward scattering ratio is maximum and most of the radiation is emitted into one strong crescent-shaped lobe pointing away from the excitation position (same data as in Fig. 2a ). Figure 5: Multipolar decomposition. Normalized experimental CL radiation patterns (row ( a )) and numerically fitted theoretical patterns (row ( b )) for a D =180 nm Au disk excited on the ‘left’ side for λ 0 =400–600 nm. The patterns are a result of the coherent interference of five multipole components. The theoretical radiation patterns for the individual components are plotted in row ( c ) for λ 0 =500 nm for a source placed 40 nm above a silicon substrate. Below each pattern the corresponding charge distribution is shown from two perspectives (row ( d )): on the left, a top view of the disk and on the right, a cross section of the disk in the xz plane. Full size image Multipolar decomposition Next, we derive a model for the single-disk radiation profiles. If the size of the nanodisk is much smaller than the wavelength it can accurately be described as a point dipole scatterer with a electric dipolar polarizability tensor [42] . For larger sizes higher-order multipole contributions become significant. The coupling efficiency to different moments strongly depends on the type of excitation [43] , [44] , particle shape and dielectric environment. In particular for cases where the particles have a non-spherical shape and/or are placed in an asymmetric dielectric environment like on a substrate, quantifying the contributions of the different multipoles is complex. Here we use a 3D surface integral equation method to find the relevant multipolar components for our experiment. In this full-wave method the nanodisk is discretized into triangular surface elements [45] , [46] . By locally solving Maxwell’s surface integrals for each individual element, the scattered fields for a particular type of driving field, eigenpolarizabilities, and the local density of optical states in the vicinity of a scatterer can be accurately calculated. This method recently has been successfully employed to describe the scattering properties of plasmonic split rings [47] . To simulate our experiment, we discretize the surfaces of cylindrical particles with 50, 100 and 180 nm diameters into surface elements using a radius of curvature of 5 nm to prevent numerical inaccuracies in the fields. We calculate dipolar and quadrupolar polarizabilities by exciting the structures with orthogonal sets of counter-propagating waves and decomposing the calculated scattered field into vector spherical harmonics. This allows us to represent the nanodisk by a point scatterer of which the scattering properties are described by its superpolarizability tensor (F.B.A, T.C. and A.F.K., manuscript in preparation; see also ref. 46 for details). To account for the effect of the substrate a backaction substrate-correction to the superpolarizability tensor is applied to the initial calculation. To drive the disk we place a vertical point dipole at the xy electron beam excitation positions used in the experiment, thereby mimicking the electron beam driving. For the z position of the dipole we study both 40 nm (at the half-height of the disk) and 80 nm (top of the disk). We find that for both excitation dipole heights the relevant components for edge excitation (in the x direction at ϕ =90°, 270°) are electrical dipole moments p z and p x , the magnetic component m y , and quadrupolar moments Q xz (corresponding to the Q 13 and Q 31 elements in the quadrupole tensor [48] ), and Q xy (corresponding to the Q 11 and − Q 22 elements in the tensor which is a quadrupole that is rotated 45° in the xy plane with respect to the Q 12 , Q 21 quadrupole). The angular patterns and corresponding charge distributions of these individual components are shown in the bottom panel of Fig. 5 . These are calculated using asymptotic far-field approximations for dipoles and quadrupoles in the presence of a substrate [49] , [50] , [51] . Both electrical dipole components p z and p x show the characteristic toroid shapes centred around the dipole axis. As the figure shows, the patterns deviate from a perfect toroid because of substrate interference [50] . Both of these dipole components have a significant E z component at the edge of the nanodisk and thus can be driven by a z dipole or electron beam at this position. The magnetic dipole component m y corresponds to an electrical current loop in the xz plane (indicated by the black dashed line in the schematic for m y in the bottom panel of Fig. 5 ), which also has a significant E z component at the edge of the disk. For the Q xz and Q xy quadrupoles the radiation patterns show multiple radiation lobes. These particular quadrupoles would show four radiation lobes in free space of which three are visible in the upper hemisphere for Q xz (because one lobe is oriented directly along the normal into the substrate where it can not be collected by our parabolic mirror) and all four are visible for Q xy because all lobes lie in the xy plane. Like for the dipole patterns the quadrupolar patterns are distorted relative to those in a homogeneous dielectric environment due to the presence of the reflective silicon substrate. Next, using the theoretical far fields of the relevant multipole components we decompose the experimental far-field angular radiation patterns by numerically fitting the complex amplitudes using a least-squares numerical optimization routine [44] , [52] . For the smaller disks ( D =50–100 nm) the patterns are dominated by p x and p z due to their size compared with the wavelength, so using only those components for the data-fitting yields good results (see Fig. 4c,f ). We find a ratio of | p z |/| p x | of 1.9 for λ 0 =600 nm for the D =100 nm disk, so the p z component is strongest in that case. Because of their pure dipolar character the resulting asymmetry in the angular pattern is smaller than for the larger disks. For the D =50 nm disk a toroidal ‘doughnut’ shaped pattern is observed, consistent with the emission pattern of a vertically oriented point dipole source (so a pure p z contribution) [49] , [50] . This is consistent with the spatial profile in Fig. 1c , where we observed an excitation maximum in the centre of the nanodisk. In contrast, for a D =180 nm disk all five dipolar and quadrupolar components mentioned above contribute to the observed radiation profiles. The bottom row of the top panel in Fig. 5 shows the angular patterns obtained from the numerical fits. They agree very well with the measured patterns. This demonstrates that the observed angular patterns indeed can be accurately described as the coherent superposition of the multipoles predicted by surface integral equation calculations. The absolute values of the different multipole moments are listed in Table 1 . For all fits the in-plane electrical dipole component p x is dominant as one might expect for a disk with this diameter and aspect ratio. Nevertheless in all fits there are significant contributions from the vertical electric dipole, magnetic dipole and electric quadrupoles. Table 1 Numerical fitting of multipole components. Full size table As is the case for Kerker scattering in dielectric/semiconductor nanoparticles [21] , [22] , [23] , [24] , [27] , strong directionality is expected only when the different multipole components are similar in magnitude as that allows effective interference in the far field. Evidently this condition is not met for the D =50 nm disk, where the pattern is fully dominated by p z and no beaming is observed. However, when we look at the fitted values for the D =180 nm particle especially at λ 0 =600 nm, the p x component is less dominant and there are significant multipolar contributions, leading to a weaker normal component of the radiation emission and strong asymmetric emission towards the side ( Fig. 2a ). For almost all measurements (except for D =50 nm at λ 0 =400 nm) the radiation is predominantly emitted away from the excitation point (see Fig. 2a ), so for these nanodisks there are no significant relative phase-flips of the components as function of wavelength that would lead to inversion of the directionality. Thus, the admixture of multipolar contributions that yields directionality can be controlled on one hand by particle size and shape, that is, by control of the multipole polarizabilities, and on the other hand by changing the particle driving by nanoscale changes in excitation position of a local source like the electron beam such that the structure is excited in an asymmetric way. An alternative way of achieving this driving asymmetry is by using circularly/elliptically polarized light as has been demonstrated recently in ref. 25 . In some cases it might be desirable to have a more universal unidirectionality, meaning that an antenna is designed in such a way that it emits in the same direction for a large variety of excitation conditions (even for symmetric excitations). This can be achieved by introducing an asymmetry in the nanostructure itself [26] , [28] . Also in this case, it has been shown that it is better to have larger structures with more polarizable material in order to promote the higher-order multipoles that facilitate a strong directional response. Rather than engineering either the driving or the structure to constrain the emitted patttern to a given asymmetric and directional distribution, we envision that the strong variability of directionality with excitation position can also be used advantageously. In particular, we propose that the type of position-dependent directionality as shown in this article lends itself perfectly for improving fluorescence correlation spectroscopy, for instance, where temporal correlations in fluorescence intensity can reveal the diffusion constant of single diffusing fluorophores [53] , [54] . By detecting fluorescence intensity of single molecules diffusing over the nanodisks in the Fourier plane with a quadrant photodiode for instance, one could utilize the antenna directionality to decrease the effective detection volume, thereby boosting the sensitivity. Finally, in our experiment the antennas are on a high-index substrate that on one hand helps with the generation of significant multipole moments through backaction on the nanodisks (F.B.A, T.C., A.F.K., manuscript in preparation) but also leads to large radiation losses into the substrate. These radiation losses could be minimized by for instance using a ground-plane geometry where a mirror underneath the structure ensures that all of the light is emitted into the upper hemisphere. The concepts shown in this work can directly be applied to such ground-plane antennas, which may lead to novel highly efficient directional antenna designs. In conclusion we have measured the directional emission properties of gold nanodisks as functions of size and wavelength using angle-resolved CL imaging spectroscopy. For the 50 nm diameter disks the angular pattern is toroidal, corresponding to an out-of-plane dipole resonance. For the larger disks the angular patterns are a coherent superposition of electric dipole, magnetic dipole and electric quadrupole contributions. For these disks we find that nanoscale lateral displacements of the electron beam over the nanodisk leads to drastic changes in the angular pattern. We find that off-centre excitation leads to an asymmetric radiation pattern where light is preferentially scattered in the forward direction, which is due to the complex far-field interference of different multipole moments generated in the disk. When the wavelength is large compared with the particle size the emission is dominated by electrical dipole components but when the particle size increases there are clear magnetic dipole and electric quadrupole contributions giving rise to strong directionality without the use of additional parasitic antenna elements. Our work could be utilized in the future to engineer strongly directional single-element antennae with a small spatial footprint, which could be used in a wide variety of applications. Sample fabrication We fabricated gold nanodisks on a crystalline silicon substrate using a combination of electron beam lithography, thermal evaporation and lift-off. We used a 350-nm-thick layer of ZEP520A as positive resist for electron beam lithography with a Raith E-line system. After exposure and development, a gold layer was deposited using thermal physical vapour deposition in vacuum. After lift-off in n-methylpyrollidone at 65 °C for 3 h, we obtained nanodisks on silicon with diameters ranging from 50–180 nm and a height of 80 nm. How to cite this article: Coenen, T. et al. Directional Emission from a Single Plasmonic Scatterer. Nat. Commun. 5:3250 doi: 10.1038/ncomms4250 (2014).